Three-dimensional strutted graphene grown by substrate-free sugar blowing for high-power-density supercapacitors Three-dimensional graphene architectures in the macroworld can in principle maintain all the extraordinary nanoscale properties of individual graphene flakes. However, current 3D graphene products suffer from poor electrical conductivity, low surface area and insufficient mechanical strength/elasticity; the interconnected self-supported reproducible 3D graphenes remain unavailable. Here we report a sugar-blowing approach based on a polymeric predecessor to synthesize a 3D graphene bubble network. The bubble network consists of mono- or few-layered graphitic membranes that are tightly glued, rigidly fixed and spatially scaffolded by micrometre-scale graphitic struts. Such a topological configuration provides intimate structural interconnectivities, freeway for electron/phonon transports, huge accessible surface area, as well as robust mechanical properties. The graphene network thus overcomes the drawbacks of presently available 3D graphene products and opens up a wide horizon for diverse practical usages, for example, high-power high-energy electrochemical capacitors, as highlighted in this work. Graphene, as an outstanding representative of two-dimensional (2D) crystals, offers unique physics and exciting functionalities [1] . In addition to electronic and photonic applications featuring its ‘2D crystal’ character, graphene can be used in large quantities as an adsorbent, a support or an electrode featuring its ‘new carbon’ status [2] , [3] and as a component of diverse composite materials featuring its ‘nano’ quality [4] . Unfortunately, the poor intersheet connections between isolated graphene flakes as building blocks break the continuous pathway for electron/phonon transports and severely suppress the intrinsically high conductivity and mechanical strength of individual graphene flakes [5] . The unavoidable restacking and agglomeration caused by van der Waals forces-induced adhesion in standard graphene products diminishes the accessible surface area [6] . New three-dimensional (3D) graphenes are thus calling for the accomplishment of perfect sheet-to-sheet connectivity and substantial supportability towards high performance in the massive applications. Many efforts have recently been made in relation to the 3D graphenes. Pillared graphenes [7] , [8] , graphene hybrids using physical/chemical assemblies on functional metals, oxides, polymers or carbon nanotube (CNT) connectors [5] , [6] , [9] , [10] , [11] , [12] , macroporous graphenes using self-assemblies [13] , [14] , [15] and graphene networks derived from direct-templated chemical vapour deposition (CVD) [16] , [17] have been proposed and studied. However, both graphene hybrids and macroporous graphenes still suffer from heterogeneous intersheet connections and high junction resistances. CVD-derived graphene networks have a good interconnection but do not yet have sufficient mechanical support due to the softness of pristine graphene frameworks. Moreover, the template utilization in CVD methods limits the large-scale production and leads to a high product cost (commercial price, $50 per cm 3 ). These currently available graphene products are still far from meeting the feasible and promising applications. Herein, inspired by an ancient food art of ‘blown sugar’, we develop a sugar-blowing technique to grow a 3D self-supported graphene product, named by us as strutted graphene (SG). SG consists of continuous graphitic membranes, which are homogenously connected and spatially supported by the networks of micrometre-width graphitic struts. The high electrical conductivity, surface area, mechanical strength and elasticity are thus simultaneously achieved in this SG. The facile low-cost high-throughput production with the sugar-blowing technique further enables its immediate practical utilizations. SG quality fully fits the above-mentioned large-scale applications, for example, supercapacitors. We additionally confirm the high power density of an SG-based supercapacitor due to such structural interconnectivities, hierarchical porous channels, huge accessible surface area and high mechanical and chemical stabilities. Characterization and properties of SG The obtained SG product reveals a foam-like architecture ( Fig. 1a ) packed by large polyhedral bubbles. The average diameter of the bubbles is 186 μm ( Supplementary Fig. S1 ). The struts are defined as the borders where three/four bubbles merged [18] . Graphitic struts with an average width of 3.5 μm constitute the skeletons of the bubbles and graphitic membranes are tightly anchored onto them as facets. The graphitic facets are mainly distorted pentagons, or sometimes quadrangles, hexagons and heptagons on a side of SG ( Fig. 1b ); this topology approaches a steady status having polygonal units of 5.1 edges per face in theory [19] . 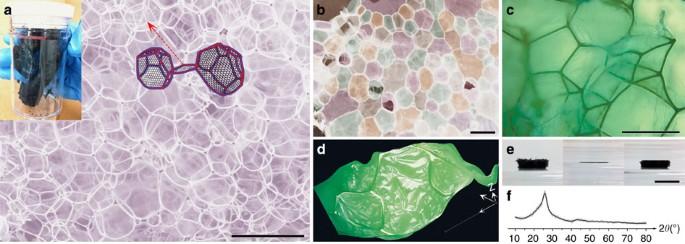Figure 1: The 3D bubble-like network of SG. (a) Scanning electron microscope (SEM) image and optical photo of a 70-mg SG piece obtained at a heating rate of 4 °C min−1. The inset is a reconstructed topology corresponding to the region marked in red for the two connected decahedron–dodecahedron bubbles faced by eight pentagons and two quadrangles, and by eight pentagons, three quadrangles and one heptagon, respectively. (b) SEM image of the flat backside of the SG product with regular arrangement of connected cells identified by artificial quilt colours. (c,d) 2D and 3D optical photos of SG networks. (e) Photos of original, compressed and recovered states of a SG specimen. (f) XRD profile of SG. Scale bars, 200 μm (ina–d) and 1 cm (ine). Figure 1: The 3D bubble-like network of SG. ( a ) Scanning electron microscope (SEM) image and optical photo of a 70-mg SG piece obtained at a heating rate of 4 °C min −1 . The inset is a reconstructed topology corresponding to the region marked in red for the two connected decahedron–dodecahedron bubbles faced by eight pentagons and two quadrangles, and by eight pentagons, three quadrangles and one heptagon, respectively. ( b ) SEM image of the flat backside of the SG product with regular arrangement of connected cells identified by artificial quilt colours. ( c , d ) 2D and 3D optical photos of SG networks. ( e ) Photos of original, compressed and recovered states of a SG specimen. ( f ) XRD profile of SG. Scale bars, 200 μm (in a – d ) and 1 cm (in e ). Full size image The interconnected struts of SG are integrated with membranes to form a unique architecture ( Fig. 1c,d ). The struts serve as connectors to conduct electrons/phonons, as fixers to resist the disintegration of graphitic membranes and as supporters to prevent agglomeration or restacking of individual graphitic membranes. SG thus has an overall high conductivity of 1 Sm −1 due to such specific structural configuration. The configuration is also beneficial for providing a smooth transfer of foreign mass within the bubble channels and for retaining the intrinsically large surface area of graphenes. The integrated architecture further determines robust mechanics of SG, although the product possesses an ultralow density of 3.0 mg cm −3 comparable to a carbon aerogel. The ultralight SG exhibits high elasticity under compression tests ( Fig. 1e ); such behaviours are similar to a graphene-based cellular monolith [20] , cork and other elastomeric foams [21] . SG can recover even under a compression to 80% ( Supplementary Fig. S2 ). The highly reversible resilience without collapse indicates the self-supporting robust structural integrity. This is further confirmed by a remarkable conductivity of 0.6 Sm −1 sustained after a heavy compression to 80%. The robust structure contributes to high tolerance/endurance with a reliable large surface area to further mechanical processing in practical applications without requirements for an additional protection. SG is a highly graphitized product. It exhibits high crystalline degree with a strong (002) peak locating at 26.0° in the X-ray diffraction (XRD) pattern ( Fig. 1f ). The broadening of this peak indicates the downsized dimensions of graphitic crystals along the [002] directions, which are estimated as 2.7 nm according to Scherrer equation. The SG has hierarchical porous structures at different scales, that is, bubbles, ripples and concaves. The bubbles are circumscribed by graphitic membranes joined onto graphitic struts. The spacious graphitic membranes are not flat but are full of dune-like ripples with an average size of 12 nm ( Fig. 2a,b ). Spontaneous and stress-induced thermodynamic relaxation of the polymer precursors in the present sugar blowing might account for these ripples, which are as fashionable as the bumps of a monolayer graphene with a 1-nm amplitude attributed to intrinsic and/or impurity-caused thermodynamic fluctuations [22] , [23] . The ripples contribute to resisting the restacking of overlapped graphenes to keep the large surface area of graphene products [24] . In addition, some concaves with an average size of 4 nm are attached on graphitic surfaces, which are encircled by (002) graphitic basal planes ( Supplementary Fig. S3 ). Such surface defects might result from oxidation by the surface C–O groups or residual O 2 on amorphous carbon under high-temperature annealing. They introduce abundant edges, that is, transverse sections of graphitic basal layers, beneficial to the specific adsorption and achieving a high surface area. 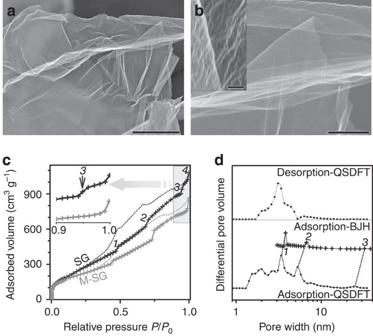Figure 2: Rippling few-layered graphene membranes and high surface area of SG. (a,b) Scanning electron microscope (SEM) images of a broken few-layered graphene membrane linked by its strut and the magnified surface with many ripples. Scale bars, 10 μm (ina), 1 μm (inb) and 200 nm (in inset ofb). (c) N2adsorption/desorption isotherms of SG and M-SG, with a particularly enlarged inset at 0.95P/P0. Numbers1–4indicate four condensations. (d) Corresponding pore-size distributions according to Barret–Joyner–Halenda (BJH) and quenched solid density function theory (QSDFT) calculation/simulation. Figure 2: Rippling few-layered graphene membranes and high surface area of SG. ( a , b ) Scanning electron microscope (SEM) images of a broken few-layered graphene membrane linked by its strut and the magnified surface with many ripples. Scale bars, 10 μm (in a ), 1 μm (in b ) and 200 nm (in inset of b ). ( c ) N 2 adsorption/desorption isotherms of SG and M-SG, with a particularly enlarged inset at 0.95 P / P 0 . Numbers 1 – 4 indicate four condensations. ( d ) Corresponding pore-size distributions according to Barret–Joyner–Halenda (BJH) and quenched solid density function theory (QSDFT) calculation/simulation. Full size image The diverse porous structures were further characterized by N 2 adsorption/desorption tests ( Fig. 2c ). SG behaves close to the type IV isotherm having four steep condensations on the adsorption part. The first three ones correspond to ‘pores’ with widths of 4, 7 and 30 nm according to Barret–Joyner–Halenda theory ( Fig. 2d ). The ‘pore’ dimensions located at condensations 1 and 2 are just consistent with the above-mentioned concaves and ripples, respectively. The steep condensation 3 around 0.95 P / P 0 results from some high-curvature regions inside the bubble cavities of SG. This condensation clearly disappeared for the milled SG (M-SG) in which the bubble structures were destroyed by heavy milling. These three structures are attributed to high-order specific morphologies mainly relevant to graphitic membranes, which can be considered as ‘mesopores’. The condensation 4 relates with the unsaturated adsorption at macroporous bubble cavities of SG or secondary piled slits of M-SG. Pore distributions based on quenched solid density function theory are similar, except a slight downshift compared with the Barret–Joyner–Halenda results. The ‘pores’ on different scales are nested and may cause the temporary locking of liquid N 2 and delayed evaporation in the desorption isotherm, which thus resembles type H3 hysteresis loops. The ‘mesoporous’ structures and supporting effect of SG struts result in a high specific surface area (SSA) of 1,005 m 2 g −1 . This is larger than for the unsupported graphene products, because the high intrinsic SSA of graphenes is always suppressed by severe agglomeration or flake restacking [25] . By contrast, M-SG without such supporting effect has a much low SSA of 780 m 2 g −1 . Moreover, the contribution fraction of micropores to the SSA and specific pore volume of SG is minor, around zero, as evidenced by a t -plot analysis. The ‘mesopores’ contribute to 55% of SSA; macroporous bubbles and external surfaces contribute with a notable fraction of 28% according to quenched solid density function theory ( Supplementary Fig. S4 and Supplementary Table S1 ). As a result, the high SSA derived from ‘mesopores’ and macroporous structures can facilitate intense and quick charge storage/release in SG electrodes for supercapacitor devices. The graphitic membranes of SG are mainly large-area, ultrathin, high-quality mono-/few-layered graphenes and some multilayered graphite sheets. A representative spacious membrane with a lateral size of ~100 μm is transferred on substrates ( Fig. 3a ). Atomic force microscopy reveals its small thickness of 2.2 nm, that is, six graphitic layers, as shown in Fig. 3b . The mono/few layers of ultrathin graphene membranes are also depicted in Fig. 3c . The small thickness is consistent with the XRD results. The sp 2 -hybridized level of such mono-/few-layered graphene membranes is nearly perfect; the fraction of sp 2 /( sp 2 + sp 3 ), by analysing the electron energy-loss spectroscopy profile [26] , is 99%, which well matches the standard graphite ( Fig. 3d ). Raman spectrum further reflects high graphitization degree of mono-/few-layered graphene membranes ( Fig. 3e ). A strong 2D peak with a narrow full width at a half maximum of 48 cm −1 features a well-graphitized double-layered graphene [27] . The high graphitization status of few-layered graphene membranes was also verified by the electron diffraction and the high conductivity of 20,000 Sm −1 ( Supplementary Fig. S5 ). This figure is close to that of graphite and is higher than ~7,000 Sm −1 of a typical reduced graphene oxide (RGO, the only graphene product available in ton quantity). 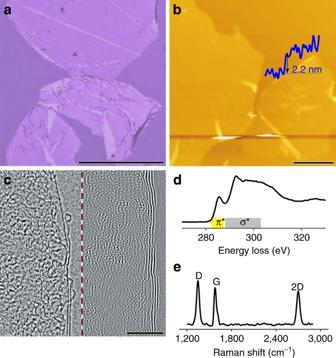Figure 3: Ultrathin high-graphitized few-layered graphene membranes. (a) Optical image of a large few-layered graphene membrane on a SiO2/Si substrate taken from SG obtained at a 4 °C min−1heating rate. Scale bar, 100 μm. (b) Atomic force microscopy image of an individual few-layered graphene membrane (the inset is a cross-section height profile). Scale bar, 5 μm. (c) High-resolution transmission electron microscopy images of a one- to two-layered graphene (left), and a three- to four-layered graphene (right). Scale bar, 5 nm. (d,e) Electron energy-loss spectroscopy profile and Raman spectrum of few-layered graphene membranes. Figure 3: Ultrathin high-graphitized few-layered graphene membranes. ( a ) Optical image of a large few-layered graphene membrane on a SiO 2 /Si substrate taken from SG obtained at a 4 °C min −1 heating rate. Scale bar, 100 μm. ( b ) Atomic force microscopy image of an individual few-layered graphene membrane (the inset is a cross-section height profile). Scale bar, 5 μm. ( c ) High-resolution transmission electron microscopy images of a one- to two-layered graphene (left), and a three- to four-layered graphene (right). Scale bar, 5 nm. ( d , e ) Electron energy-loss spectroscopy profile and Raman spectrum of few-layered graphene membranes. Full size image Growth and structural regulation of SG The SG was synthesized through the controlled heating of glucose and NH 4 Cl ( Fig. 4a ). In this process, a molten syrup was gradually polymerized, whereas chemically released gases from NH 4 Cl blew glucose-derived polymers, such as melanoidin ( Supplementary Fig. S6 and Supplementary Note 1 ), into numerous large bubbles, which features the sugar blowing. The bubble walls were gradually thinned by the gas release and blowing, surface-tension-induced drainage of the polymer fluid out of the walls and elimination of small molecules from the polymers. The polymer walls were subsequently graphitized into ultrathin graphitic membranes at a high temperature. 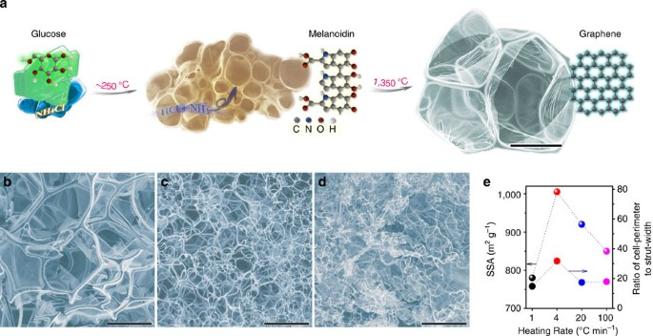Figure 4: Growth process and structural regulation of sugar-blowing production. (a) Scanning electron microscope (SEM) images of glucose (crystals marked in green) and NH4Cl (marked in blue), which were subsequently transformed to melanoidin bubbles (marked in brown) under a browning reaction; these were finally converted into the SG containing graphitic membranes and struts (marked in gray). The artificial melanoidin macromolecule structure is proposed with features of indole and catechol according toSupplementary Note 1. The heating rate is 4 °C min−1. Scale bar, 50 μm. (b–d) SEM images of the SG products grown at the heating rates of 1, 20 and 100 °C min−1, respectively. Scale bars, 200 μm. (e) Changes of SSA and ratio of cell perimeter to strut width versus heating rates. Figure 4: Growth process and structural regulation of sugar-blowing production. ( a ) Scanning electron microscope (SEM) images of glucose (crystals marked in green) and NH 4 Cl (marked in blue), which were subsequently transformed to melanoidin bubbles (marked in brown) under a browning reaction; these were finally converted into the SG containing graphitic membranes and struts (marked in gray). The artificial melanoidin macromolecule structure is proposed with features of indole and catechol according to Supplementary Note 1 . The heating rate is 4 °C min −1 . Scale bar, 50 μm. ( b – d ) SEM images of the SG products grown at the heating rates of 1, 20 and 100 °C min −1 , respectively. Scale bars, 200 μm. ( e ) Changes of SSA and ratio of cell perimeter to strut width versus heating rates. Full size image On the basis of the understanding of sugar blowing, we synthesized different SG products by regulating the heating rates ( Fig. 4b–d and Supplementary Fig. S7 ). Both cell size and strut width decrease with an increase of heating rate and the bubbles become more distorted at a faster heating rate. The ratio of cell perimeter to strut width reflects the fraction of graphitic membranes in the entire foam and thus verifies the quality of SG. The ratio is highest at a heating rate of 4 °C min −1 , indicating the optimized SG architecture; this is consistent with the SSA conclusive data from N 2 adsorption ( Fig. 4e ). The optimized SG has a topological structure of an 80-μm cell size and a 186-μm bubble diameter in average, as discussed above. The key point in the sugar blowing, that is, the match between ammonium salt decomposition and glucose polymerization, is crucial to produce the highest-quality SG, whereas the mismatched ammonia-release of (NH 4 ) 2 SO 4 , (NH 4 ) 2 CO 3 or urea with the curing of glucose-derived polymers resulted in poor-quality products ( Supplementary Fig. S8 and Supplementary Note 2 ). The best-quality SG can display exciting 2D graphene properties and functionalities more and thus has been applied by us to construct SG-based supercapacitors. SG-based supercapacitors The specific topological configuration of SG enables its high performance in an electrical double-layer capacitor (EDLC). A supercapacitor using SG obtained at 4 °C min −1 was examined by a two-electrode system in an H 2 SO 4 electrolyte. During constant-current discharging, the nearly linear voltage profiles closely approach an ideal capacitor ( Fig. 5a ). The capacitance is as high as 250 F g −1 at 1 A g −1 and slowly decreases to 130 F g −1 at a high current of 100 A g −1 ( Fig. 5b ). While testing M-SG-based supercapacitors, the initial voltage drop is much larger than in the case of SG-based ones, which determines a large internal resistance of M-SG. M-SG electrodes only demonstrate 41 F g −1 at 100 A g −1 , much smaller figures than that of SG. Commercial graphene platelets (GP) and activated carbon (AC) materials also exhibit weaker supercapacitor performances compared with SG. This was further confirmed by the alternating-current tests ( Fig. 5c ). At high frequencies, SG-based supercapacitors have a slower capacitance decay than those of M-SG ones, as indicated by the slopes of fitting lines. The SG-based supercapacitors present high average-power density and energy density ( Fig. 5d ). The high available average-power density of SG-based supercapacitors is close to an aluminum electrolytic capacitor; this is higher than for the EDLCs of CNT/graphene sponge [28] , graphene hybrid [29] , 3D RGO hydrogel [30] , [31] and a pseudocapacitor of 3D oxides [32] . 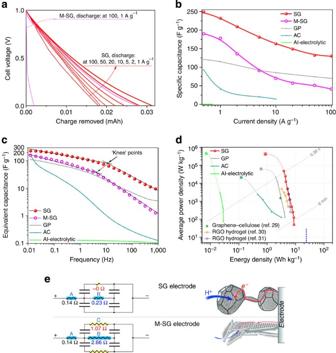Figure 5: Supercapacitor performance of SG electrodes. (a) Nearly ideal capacitor behaviours of SG electrodes under galvanostatic discharges at marked currents. (b) Correlation of specific capacitances with discharge currents of SG electrodes compared with M-SG, GP, AC and Al-electrolytic capacitor (denoted as Al-electrolytic). (c) Equivalent capacitances calculated from the frequency response analysis based on a serial RC model. The straight lines are the fitted ones as discussed inSupplementary Note 3. (d) Ragone plots of the average-power density versus energy density of supercapacitors. Previously reported 3D-graphene-based supercapacitors are plotted for comparison. The Al-electrolytic capacitor was operated in an organic system with a 25-V voltage. The blue vertical line is the theoretical upper bound of graphene–H2SO4system, that is, maximal capacitance 710 F g−1(Supplementary Table S4). The points in square frames are a half of the calculated maximum powers according to the alternating-current effective series resistance (see equations 8 and 9). (e) Equivalent circuits (left) and schematic models (right) showing easy ion diffusion and minimized inner contacts for an SG electrode compared with the M-SG one.RAandRBindicate ionic resistors of bulk electrolytes and electrolytes inside electrode pores, respectively.RCreflects contact resistors within electrode materials (see more inSupplementary Table S2andSupplementary Note 3). Figure 5: Supercapacitor performance of SG electrodes. ( a ) Nearly ideal capacitor behaviours of SG electrodes under galvanostatic discharges at marked currents. ( b ) Correlation of specific capacitances with discharge currents of SG electrodes compared with M-SG, GP, AC and Al-electrolytic capacitor (denoted as Al-electrolytic). ( c ) Equivalent capacitances calculated from the frequency response analysis based on a serial RC model. The straight lines are the fitted ones as discussed in Supplementary Note 3 . ( d ) Ragone plots of the average-power density versus energy density of supercapacitors. Previously reported 3D-graphene-based supercapacitors are plotted for comparison. The Al-electrolytic capacitor was operated in an organic system with a 25-V voltage. The blue vertical line is the theoretical upper bound of graphene–H 2 SO 4 system, that is, maximal capacitance 710 F g −1 ( Supplementary Table S4 ). The points in square frames are a half of the calculated maximum powers according to the alternating-current effective series resistance (see equations 8 and 9). ( e ) Equivalent circuits (left) and schematic models (right) showing easy ion diffusion and minimized inner contacts for an SG electrode compared with the M-SG one. R A and R B indicate ionic resistors of bulk electrolytes and electrolytes inside electrode pores, respectively. R C reflects contact resistors within electrode materials (see more in Supplementary Table S2 and Supplementary Note 3 ). Full size image The excellent performances of SG electrodes are determined by three factors ( Fig. 5e ): (i) total SG porosity is 99.85% as calculated from its apparent density; bubble cavities take the most SG volume. The cavities are connected by breaches and opened cells to form pathways for the smooth ion migration; inside the cavities the channel resistance is notated as R B . This resistance is only 0.23 Ω for SG electrodes, whereas it increases to 2.66 Ω for M-SG electrodes ( Supplementary Fig. S9 , Supplementary Table S2 , and Supplementary Note 3 ). This reflects the large diffusion drag and the exhaustion of ions within the confined piled pores and a narrow neck-like channel of the M-SG. The capacitance decay at the high-frequency domain can be attributed to distributed charge storage in electrode pores (equivalent to resistor-capacitor networks in a transmission-line model) and/or ion diffusion control [33] . The suppressed diffusion in M-SG electrodes thus causes the steep capacitance decay and a small capacitance at 10 3 Hz. By contrast, the surfaces of SG can be readily accessed without a diffusion limit, which guarantees a large capacitance at extremely high currents/frequencies. (ii) A natural, nearly perfect electron freeway is provided by the interconnected struts and by joined graphitic membranes in SG. The inner contact resistance of SG electrodes thus is nearly zero, but it is 1.07 Ω for M-SG electrodes owing to many intersheet contacts ( Supplementary Table S2 ). Such large resistance results in a larger initial voltage drop and smaller available output power and energy; it also contributes to the earlier appearance of ‘knee’ inflexion at a lower frequency for M-SG electrodes, because such contact resistors are distributed and coupled with EDLC networks. The frequency at the ‘knee’ point is the upper limit for utilizing most of cavity and pore surfaces below which the capacitance approaches its intrinsic value. The SG electrodes oppositely have a higher ‘knee’ frequency (11 Hz), a lower capacitance-cutoff impedance (~0.4 Ω) and a higher characteristic frequency (9.6 Hz; see Fig. 5d and Supplementary Fig. S10 ). (iii) In M-SG, individual graphitic flakes may easily agglomerate and restack into multilayered structures. This results in inaccessible surfaces and the capacitance loss [34] , [35] . On the contrary, the graphitic membranes in SG are attached and rigidly fixed on their partners, the strut networks. This avoids the agglomeration and leads to the highest capacitance. SG electrodes also perform better than the GP ones and much better than microporous AC ones due to the similar factors. Their power density and energy density are thus undoubtedly outstanding compared with other EDLCs. The maximum power density is widely accepted as a fundamental property of supercapacitors. The maximum power density of SG, achieving 893 kW g −1 at 100 A g −1 , is further compared with other materials in Supplementary Fig. S11a and Supplementary Table S3 , showing one-to-two orders of magnitude higher values than those for all previously reported 3D graphenes [16] , [36] , [37] , [38] . The high power density not only implies quick charging completed within a few seconds but also presumes the huge available energy output within the limited time. The superfast available charging process illuminates an amazing future in ‘flash charging’ of portable electronics, quick startup of electric vehicles and electromagnetic launching of aircrafts. The developed sugar-blowing technique can reliably produce SG using many common precursors such as glucose and kitchen-use sugar ( Supplementary Fig. S12 ). It therefore provides a universal pathway and opens a new window for the creation of 3D graphene analogues. In addition, it should be considered as a new member of the family of synthetic protocols of 3D graphene. The facile sugar-blowing method stands out of many previous routes for making 3D graphenes, such as hydrothermal method [13] , [39] , [40] , cryodesiccation [15] , [41] , breath-figure method [14] and CVD [16] , [17] , [42] . The produced SG normally possesses larger surface area than graphene papers [43] , higher conductivity than widely studied RGO hydrogels and stronger mechanical endurance than CVD-derived graphene foams. Moreover, the high-yield sugar-blowing route makes the production of SG scalable, up to kilogram or even ton levels. Massive SG has been produced at a yield of 16±5 wt% related to a raw glucose following the designed sugar-blowing method. The product costs only $0.5 per gram referring to our laboratory-scale synthesis, in contrary to much more expensive other 3D graphene products. The abundant production of SG together with its unique structural characteristics enlightens its wide and promising potentials. The mono-/few-layered graphene membranes of SG have the high graphitization degree. During sugar blowing, the walls of sugar-derived polymer bubbles are thinned down to ~ 20 nm by the expansion of released gases and surface drainage. Meanwhile, the elastic, highly elastic and viscous interior stresses are induced along the polymer walls of bubbles. As both ultrathin thickness and interior stress are beneficial to orient polymer molecules [44] , the present bubble walls possess highly oriented arrangement of polymer molecules. The graphitization on such thin-oriented polymeric predecessors is easier than the conventional graphitization of a bulk carbon resource or carbon films/fibres at micrometre level [45] , because the energy used for the parallel arrangement of (002) graphitic layers becomes much lower in case of an oriented predecessor [46] , [47] . Hence, the well-graphitized graphitic membranes are formed. The graphitization approach of sugar blowing is clearly different from all previous methods of graphene syntheses, such as diverse exfoliations [48] , [49] , [50] , CVD [51] , solvothermal, organic synthesis [34] , [52] and substrate-assistant/catalytic graphitization [53] , [54] , [55] . It illuminates a new graphene synthesis mechanism calling for extensive researches. The structural regulation of SG was realized through modifying heating rates. The heating rate acts through the matching relation between the gas release and polymer curing owing to kinetics factors, including decomposition of NH 4 Cl, diffusion of gas, nucleation and growth of bubbles. This control is consistent with the experience in traditional polymer foaming. Furthermore, some rheology courses such as drainage, rupture and coalescence of bubbles also influence the bubbling process. In the bubble growth, the volume expansion is forced by gas release. The applied energy trades with viscous flow and increasing surface area of bubbles. More effectively utilized gas can cause a larger viscous deformation and thus larger bubbles, giving the same acting trend in line with the kinetic factors ( Supplementary Note 2 ). In bubble dilation, the interior stress strongly depends on the heating rates. A higher heating rate can substantially lead to the higher elastic interior stresses. This results in stronger shrinkage/distortion of bubbles when NH 4 Cl exhausts, as observed in Figs 1a and 4b–d . The drainage is caused by surface tension. Smaller curvature radius at Plateau borders results in the smaller pressure compared with bubble walls, and thus a Laplace force causes continuous drainage of the intralamellar fluid into the borders, that is, gradual thinning of bubble walls. This mass transfer depends on surface viscosity and time [56] . A slow heating process gives rise to more fluid flowing into borders and thus thicker struts, as shown in Figs 1a and 4b–d and Supplementary Fig. S7c . One of the most important purposes to develop the 3D graphene subdiscipline is to reach the high power density of its supercapacitors. For example, they can be combined with a battery for power pulse output with a low overall internal resistance and long lifetime. The power density of rechargeable batteries is normally <500 W kg −1 ; micropore-type supercapacitors have the power density of 10 2 –10 4 W kg −1 ; thick-layer graphene supercapacitors have the power density of 10 3 –10 4 W kg −1 (ref. 57 ). These relatively low power densities are limited by the block effect of narrow channels to ion migration and the resistance of discontinuous matrix to electron transport. The 3D carbon-based supercapacitors, such as CNT networks [58] and 3D graphenes, do not have the above-mentioned disadvantages in theory and can have increased power density. Our SG undoubtedly satisfies the three main requirements for porous electrodes: (i) sufficiently connected cavities/channels providing an electrolyte pathway to maximize ionic conductivity and to have a free access to the inner surface; (ii) the minimal contact resistance between blocks building the porous electrodes; and (iii) a large SSA and the robust mechanical structure. The SG thus nicely functions in supercapacitors with a high maximum power density close to 10 6 W kg −1 resulting from the former two advantages. A relatively high usable energy density is also achieved by merging all three mentioned factors. In addition, a maximum volumetric power density of 27 kW L −1 of our supercapacitors was achieved after appropriate compression of SG (denoted as C-SG, see Supplementary Fig. S11b,c ). The volume of C-SG decreased after compression, whereas its electronic and ionic resistances did not increase much; these features determined a higher maximum volumetric power density than the SG ones [59] , [60] . Furthermore, these SG electrodes have no restrictions for the further scaled-up fabrication due to their interconnected architectures, whereas analogous characteristics of normal graphene-based supercapacitors decay with scaling up the loading mass/thickness on an electrode [57] , [61] . In summary, we have developed a sugar-blowing approach to effectively synthesize a 3D graphene product, namely SG, which is made of graphitic membranes tightly connected and supported by robust graphitic microstruts. The developed reliable and scalable synthetic protocol is envisaged to become a general path for the synthesis of 3D graphene analogues, especially meaningful BC x N graphenes. The produced abundant SG enables many graphene-related applications as supports, catalysts, sorbents, hydrogen reservoirs, gas sensors, air filters, sound absorbers for substituting current porous carbons and as the nano-fillers of functional nanocomposites. The selected example, SG-based supercapacitors, exhibit very high power densities. The robust 3D topology of SG further allows avoiding disintegration and performance decay in any scaled-up device fabrication process. Synthesis of SG Typically, 10 g glucose was mixed with 10 g ammonium salts (NH 4 Cl), which was then heated under a desired heating rate (4 °C min −1 was recommended) and finally treated at 1,350 °C for 3 h under Ar atmosphere in a tube furnace (50 cm length by 5 cm diameter). A black foam-like product, that is, SG, was collected. White granulated sugar (a kitchen-use sugar from Nissin-Sugar Co.) was also used to replace glucose to grow SG. Characterizations of SG The morphologies of SG were visualized by scanning electron microscopy (Hitachi S-4800), high-resolution transmission electron microscopy (JEOL JEM-3000F), atomic force microscopy (JEOL JSPM-5200) and optical microscopy (Keyence VHX-900). The structures were characterized by electron diffraction and energy-loss spectroscopy (attachments of JEOL JEM-3100FEF with an Omega Filter), XRD (Rigaku Ultima III with Cu Kα radiation), Raman spectroscopy (a Kr-Ar ion laser at 514 nm produced by Spectra-Physics Beamlok 2060-RS laser combining Symphony CCD-1LS detection system) and Fourier transform infrared spectroscopy (Thermo Nicolet 4700). The thermal analysis was done using thermogravimetric and derivative thermogravimetric (Rigaku Thermo plus TG 8120) methods, as well as differential scanning calorimetry (Rigaku Thermo plus EVO DSC8230). The nitrogen adsorption–desorption measurements were carried out at a liquid nitrogen temperature on a Quantachrome Autosorb-1. Brunauer–Emmett–Teller surface area was estimated over a relative pressure range of 0.05–0.3. The conductivity of individual few-layered graphene membranes was analysed within a field effect transistor configuration using a semiconductor parameter analyser (Keithley 4200-SCS). Supercapacitors based on SG The symmetric supercapacitors were fabricated using two electrodes made of diverse 1.0 mg active materials: SG, M-SG, commercial GP (from ACS Material LLC) and AC (charcoal activated, Merck Chemicals Co.), respectively. SG-based electrodes were made through placing SG foam-like blocks with designed shape onto steel collectors, to which surfaces a thin-layered binder of polyvinylidene fluoride was in advance applied; tetrafluoroethylene were further used to fix the SG blocks to collectors. If a 1 MPa pressure force was applied to the SG/collectors when drying them, the C-SG electrodes were thus prepared. The other active materials were tested here for comparison purposes (SG was in advance milled into powders in a mortar as a control denoted as M-SG). They were typically mixed with tetrafluoroethylene by 10:1 ratio in water solutions; the concentrated mixtures were then pasted onto collectors and dried at 60 °C. The electrochemical examinations of the supercapacitors, including chronopotentiometry, cyclic voltammetry and electrochemical impedance spectrometry were conducted in a 1 M H 2 SO 4 electrolyte by an electrochemical workstation (Solartron 1280B). The galvanostatic discharge at 100 A g −1 of M-SG supercapacitors was measured by an electrochemical analyser (HJ1001SD8, OKUTO DENKO Co.). An Al-electrolytic capacitor of 25-V/4.7-μF (Su’scon Co.) was also tested for comparison, in which two Al foils were 16 mg in weight and the dry packaging materials were 140 mg. The gravimetric capacitance normalized on one electrode ( C g ) was calculated from galvanostatic constant-current discharging measurements in two-electrode systems using: where I cons is the constant current in discharging (or steady current in cyclic voltammetry curves), m is the total mass of both electrodes and d V /d t is the slope of discharge curve. The current density is normalized with respect to the mass loaded on an electrode. The direct-current equivalent internal resistance of the cell can be obtained in continuous charging/discharging by: where V drop is the initial Ohmic voltage drop of the cell at the beginning of the discharge, which is obtained through extrapolating the voltage–time curve back to zero time; such calculated apparent equivalent internal resistance may be larger than the true value at a low current due to the additional contribution of self-discharge to voltage drop. This is further used for the calculation of discharge energy densities of two electrodes E s , average-power densities of two electrodes P s and maximum constant-current discharge power densities of two electrodes P s,max-DC by using the formulas [33] , [62] : where V open-circuit is the open-circuit voltage of the supercapacitor after being completely charged to 1 V; V max is the applied voltage of the cell at maximum, 1 V for an aqueous system, here the difference between open circuit voltage and maximal voltage is small and ignored according to our measurements; and Δ t is the discharge time of the cell. The similar calculations are normalized to the volumes of active materials again. The volumetric energy densities of two electrodes E V and maximum volumetric power densities of two electrodes P V,max are determined according to: where V AM is the volume of active materials on both electrodes. The effective series resistance R ESR of the cell, determined from the x -intercept of the Nyquist plots of frequency analysis, is also used to predict the maximum power densities of two electrodes and corresponding energy densities of two electrodes by: Note that the points ( E s, at maximum power , 1/2 P s, max-AC ) were plotted into Fig. 5d to match the definition of average-power density of the vertical axis. The alternating-current equivalent capacitance normalized on one electrode ( C eq ) at frequency f was calculated from the imaginary component of the impedance ( Z′′ ) of the cell using a series-RC circuit model by: How to cite this article: Wang, X. et al . Three-dimensional strutted graphene grown by substrate-free sugar blowing for high-power-density supercapacitors. Nat. Comm. 4:2905 doi: 10.1038/ncomms3905 (2013).